The 19S proteasome subunit Rpt3 regulates distribution of CENP-A by associating with centromeric chromatin CENP-A, a variant of histone H3, is incorporated into centromeric chromatin and plays a role during kinetochore establishment. In fission yeast, the localization of CENP-A is limited to a region spanning 10–20 kb of the core domain of the centromere. Here, we report a mutant ( rpt3-1 ) in which this region is expanded to 40–70 kb. Likely due to abnormal distribution of CENP-A, this mutant exhibits chromosome instability and enhanced gene silencing. Interestingly, the rpt3 + gene encodes a subunit of the 19S proteasome, which localizes to the nuclear membrane. Although Rpt3 associates with centromeric chromatin, the mutant protein has lost this localization. A loss of the cut8 + gene encoding an anchor of the proteasome to the nuclear membrane causes similar phenotypes as observed in the rpt3-1 mutant. Thus, we propose that the proteasome (or its subcomplex) associates with centromeric chromatin and regulates distribution of CENP-A. Centromere chromatin is characteristic for the presence of CENP-A, a variant of histone H3. Chromatin composed of CENP-A plays a key role as the site of kinetochore formation and therefore is important for accurate chromosome segregation [1] , [2] , [3] , [4] , [5] . Distribution of CENP-A must be strictly regulated so that the size and number of the centromere per chromosome are maintained properly through the generations. Deviation in the size of a centromere would result in formation of an abnormally sized kinetochore, which could not interact with the spindle properly [6] . In most eukaryotes, with the exception of holocentric species [7] , each chromosome contains a single distinct centromere. A chromosome experimentally forced to have an additional centromere undergoes successive rounds of anaphase bridge formation and breakage in budding yeast and fly [8] , [9] , [10] . In fission yeast dicentric chromosomes trigger a cell cycle arrest imposed by DNA damage and replication checkpoints [11] . Nonetheless, CENP-A has a potential to be incorporated into noncentromeric chromatin. Overexpression of CENP-A results in promiscuous incorporation throughout the genome [12] , [13] , [14] , [15] , [16] . It has also been shown that CENP-A is rapidly recruited to double-strand breaks in DNA [17] . De novo formation of a kinetochore on a noncentromere locus, known as ‘neocentromere’ [18] , [19] , [20] , [21] suggest that CENP-A incorporated into noncentromeric chromatin could mature to the functional centromere. To maintain the normal karyotype and function of the centromere, accurate distribution of CENP-A would be maintained by collaboration between mechanisms to incorporate CENP-A into centromeric chromatin and those to eliminate CENP-A incorporated inappropriately. Although extensive studies have elucidated mechanisms of CENP-A incorporation [22] , [23] , [24] , our understanding of mechanisms of elimination of CENP-A has still been limited. In this study using the fission yeast Schizosaccharomyces pombe as a model organism, we have attempted to investigate a mechanism for maintenance of proper distribution of CENP-A. Through a genetic screen for mutants unable to maintain proper distribution of CENP-A, we have isolated a mutant ( rpt3-1 ) in the gene encoding a subunit of 19S regulatory particle (RP) of the 26S proteasome. Our analysis has indicated that distribution of CENP-A is maintained by the proteasome or its subcomplex that associates with the centromeric chromatin at the nuclear membrane. Isolation of rpt3-1 mutant We reasoned that a mutant unable to maintain proper distribution of CENP-A would be sensitive to expression of CENP-A at a higher level. A strain ectopically expressing Cnp1 (a fission yeast homologue of CENP-A) tagged with GFP (green fluorescent protein) from an inducible promoter was chemically mutagenized. The survivors were screened with the following two criteria; 1) to exhibit a temperature sensitivity upon induction of GFP-Cnp1, and 2) to exhibit abnormal distribution of GFP-Cnp1 in the nucleus. As shown in Supplementary Fig. 1a , one of the mutants identified through the screen, which was named rpt3-1 , became temperature sensitive upon induction of ectopic expression of GFP-Cnp1, but not histone GFP-H3, demonstrating the sensitivity of the mutant specific to Cnp1. Microscopic observation revealed that the fluorescent signal from ectopically expressed GFP-Cnp1, which appeared a discrete speckle in most of the wild-type cells due to clustering of three centromeres adjacent to the spindle pole body, SPB [25] , was found as several patches in the mutant ( Supplementary Fig. 1b,c ). While the GFP-patches associated with SPB likely represented Cnp1 incorporated in centromere(s), the origin of other patches remained to be identified. We speculated that the three centromeres no longer clustered in the rpt3-1 mutant, or these patches represented Cnp1 stochastically incorporated into one ore more of noncentromere regions. In fission yeast, each centromere contains a central domain ( cnt ) that is flanked by innermost repeats ( imr ), which together provide the core of kinetochore formation. This core domain is surrounded by arrays of outer repeats ( otr ) [26] , [27] . Previous studies showed that Cnp1 is preferentially incorporated into cnt and imr , but poorly into otr [5] . A genome-wide analysis by chromatin immunoprecipitation (ChIP)-on-chip revealed that GFP-Cnp1 expressed ectopically was incorporated cnt and imr as well as otr in the mutant ( Fig. 1a,b and Supplementary Fig. 2a ). As a result, Cnp1-positive regions, which normally was limited within 10–20 kb in the wild-type strain, span 40–70 kb in the centromeric chromatin of the mutant. In addition, GFP-Cnp1 in the mutant was incorporated into rRNA gene(s) ( Supplementary Fig. 3 ). These results suggested that the rpt3-1 mutant was unable to maintain proper distribution of GFP-Cnp1 expressed ectopically. 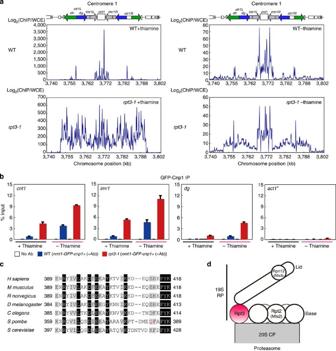Figure 1: Mapping ofrpt3-1mutation. (a,b) ChIP-on-chip analysis was performed once with samples prepared from the strains grown at 33 °C with or without thiamine. Distribution of Cnp1 around centromere 1 in the wild-type strain (WT) and therpt3-1mutant (rpt3-1) is shown ina. The results of the ChIP-on-chip analysis was further confirmed by ChIP–qPCR. Data represent the mean±s.e.m. (n=2). (b). Distribution of Cnp1 around centromere 2 and 3 is shown inSupplementary Fig. 2. (c) Partial amino-acid sequences of Rpt3 from seven species are aligned. The mutation site in the fission yeast Rpt3-1 is shown in red. (d) Proteins investigated in this study (Rpt3, Rpt2/Mts2 and Rpn12/Mts3) are shown on a schematic illustration of the 26S proteasome. Figure 1: Mapping of rpt3-1 mutation. ( a , b ) ChIP-on-chip analysis was performed once with samples prepared from the strains grown at 33 °C with or without thiamine. Distribution of Cnp1 around centromere 1 in the wild-type strain (WT) and the rpt3-1 mutant ( rpt3-1 ) is shown in a . The results of the ChIP-on-chip analysis was further confirmed by ChIP–qPCR. Data represent the mean±s.e.m. ( n =2). ( b ). Distribution of Cnp1 around centromere 2 and 3 is shown in Supplementary Fig. 2 . ( c ) Partial amino-acid sequences of Rpt3 from seven species are aligned. The mutation site in the fission yeast Rpt3-1 is shown in red. ( d ) Proteins investigated in this study (Rpt3, Rpt2/Mts2 and Rpn12/Mts3) are shown on a schematic illustration of the 26S proteasome. Full size image By using the temperature sensitivity that was dependent on overexpression of Cnp1 as a selection marker, a genomic DNA fragment complementing the temperature sensitivity was isolated from a fission yeast genomic DNA library. The integration mapping proved that this fragment originated from the rpt3 + locus encoding a subunit of 19S RP of the 26S proteasome [28] , [29] . Sequencing of the rpt3-1 mutant gene identified a nonsense mutation at Q384 of the gene ( Fig. 1c,d ). Although the mutation was mapped on a gene with a proteolytic function, the mutant could maintain the level of Cnp1 comparable with that of the wild-type cell ( Supplementary Fig. 2b ). Centromeric function of the rpt3-1 mutant Because we attempted to investigate a role of Rpt3 in maintenance of proper distribution of Cnp1 in the centromeric chromatin under physiological conditions, the experiments described below were performed with cells expressing Cnp1 tagged with 8xMyc (8xMyc-Cnp1) from the native promoter unless otherwise stated. As shown in Fig. 2a , the rpt3-1 mutant grew slightly slower than the wild-type strain at 26 and 36 °C. The level of 8xMyc-Cnp1 in the mutant was comparable with that in the wild-type strain ( Fig. 2b ). We however found by performing ChIP that the centromere contained more Cnp1 at cnt1 , imr1 and otr1 (represented by dg ) in the mutant ( Fig. 2c ). The quantitative analysis by ChIP–quantitative PCR revealed that Cnp1 in the mutant was incorporated into cnt1 more than 2-fold, imr1 1.5-fold and otr1 (represented by dg and dh ) more than 3-fold of Cnp1 in the wild-type strain ( Fig. 2d ). These results indicated that the rpt3-1 mutant could maintain the normal level of Cnp1, but not proper distribution of Cnp1 in the centromeric chromatin. 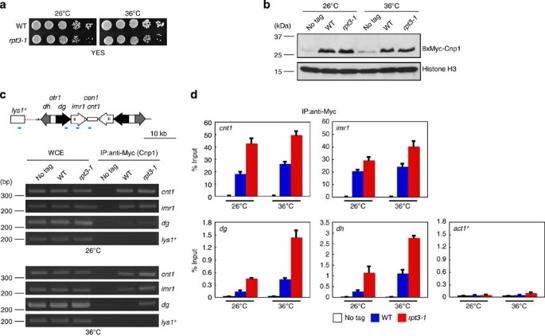Figure 2: Distribution of Cnp1 at centromere 1. (a) The wild-type strain (WT) and therpt3-1mutant (rpt3-1) were spotted on YES media and incubated at 26 or 36 °C for 3–4 days. (b) The levels of Cnp1 tagged with 8xMyc (8xMyc-Cnp1) expressed from the native promoter was examined by immublot. (c,d) Distribution of 8xMyc-Cnp1 in centromere 1 was examined by ChIP (c) and ChIP–qPCR (d). All data represent the mean±s.e.m. (n=3). The blue bars indicate the position of primers used for ChIP and ChIP–qPCR. Figure 2: Distribution of Cnp1 at centromere 1. ( a ) The wild-type strain (WT) and the rpt3-1 mutant ( rpt3-1 ) were spotted on YES media and incubated at 26 or 36 °C for 3–4 days. ( b ) The levels of Cnp1 tagged with 8xMyc (8xMyc-Cnp1) expressed from the native promoter was examined by immublot. ( c , d ) Distribution of 8xMyc-Cnp1 in centromere 1 was examined by ChIP ( c ) and ChIP–qPCR ( d ). All data represent the mean±s.e.m. ( n =3). The blue bars indicate the position of primers used for ChIP and ChIP–qPCR. Full size image It was previously shown that Cnp1 excessively incorporated into centromere chromatin affects gene silencing at the centromere [30] . Furthermore a previous study reported that gene silencing at centromeric regions became tighter in several mutants with deficiency in subunits of the 19S RP [31] . These results prompted us to investigate the gene silencing at the centromere in the rpt3-1 mutant. A previous study [31] showed that silencing of the ura4 + gene inserted at cnt1 is moderate and allows growth on 5-fluoroorotic acid (FOA) at 26 °C in a wild-type background. However, this ability is lost at 36 °C, indicating that silencing of the ura4 + gene expression within the centromere is alleviated by increased temperatures. As shown in Fig. 3a , expression of the ura4 + gene inserted at cnt domain of cen1 was severely silenced at both 26 and 36 °C. Fission yeast Swi6 (a homologue of HP1), which normally binds to otr domains [27] , [32] , is responsible for gene silencing. We therefore examine the level and distribution of Swi6 in the rpt3-1 mutant. As shown in Fig. 3c–e , although the level of Swi6 in the mutant was comparable with that of the wild-type stain, it was found at cnt1 domain. Gene silencing at imr1 and otr1 was also enhanced in the rpt3-1 mutant ( Fig. 3b ). Genetic analysis indicated that Swi6 was partially responsible for gene silencing at cnt1 in the mutant ( Fig. 3a ), and fully responsible for at imr and otr domains ( Fig. 3b ). 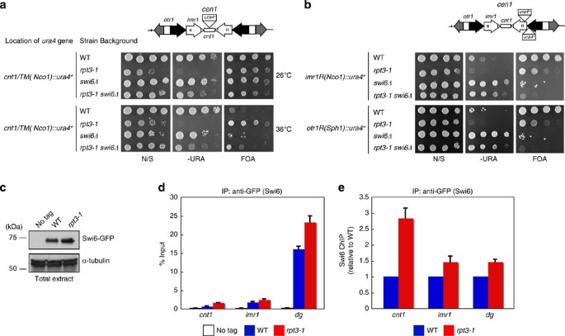Figure 3: Swi6-dependent enhancement of silencing inrpt3-1mutant. (a,b) The reporter geneura4+was integrated atcnt1(a),imr1R(b, upper panel) orotr1R(b, lower panel) and examined its expression in each strain. (c) The level of Swi6-GFP was examined by western blot. α-tubulin was used as a loading control. (d,e) The wild-type stain (WT) and therpt3-1mutant (rpt3-1) expressing Swi6 tagged with GFP from the native locus were grown at 30 °C. ChIP–qPCR was performed to examine distribution of Swi6 around centromere 1. The result is shown indas percentage of input, and ineas ratio to the wild-type strain. All data represent the mean±s.e.m. (n=3). Figure 3: Swi6-dependent enhancement of silencing in rpt3-1 mutant. ( a , b ) The reporter gene ura4 + was integrated at cnt1 ( a ), imr1R ( b , upper panel) or otr1R ( b , lower panel) and examined its expression in each strain. ( c ) The level of Swi6-GFP was examined by western blot. α-tubulin was used as a loading control. ( d , e ) The wild-type stain (WT) and the rpt3-1 mutant ( rpt3-1 ) expressing Swi6 tagged with GFP from the native locus were grown at 30 °C. ChIP–qPCR was performed to examine distribution of Swi6 around centromere 1. The result is shown in d as percentage of input, and in e as ratio to the wild-type strain. All data represent the mean±s.e.m. ( n =3). Full size image Because the above results indicated that the rpt3-1 mutation affects distribution of both Cnp1 and Swi6, it might be possible that the mutation would affect chromosome stability as well. Indeed, we found that the mini-chromosome, Ch16, was unstable in the mutant ( Table 1 ). It was previously shown that an excess amount of histone H3 competes with Cnp1 for assembly into central domains of centromeric chromatin [30] . We therefore reasoned that overexpression of histone H3 would improve the stability of the mini-chromosome in the rpt3-1 mutant if Cnp1 excessively incorporated into the centromeric chromatin were a cause of the instability. As shown in Table 2 , although overexpression of histone H3 in the wild-type strain reduced the stability of the mini-chromosome, it improved the stability in the rpt3-1 mutant. Taken together, these results would suggest that the centromeric function of the rpt3-1 mutant was disturbed due to Cnp1 excessively incorporated into the centromeric chromatin. Because improvement of the stability of the mini-chromosome is incomplete and overexpression of histone H3 can have deleterious effects on cells, future studies using alternative strategies will allow reinvestigation of the precise cause of the instability. Table 1 Stability of mini-chromosome. Full size table Table 2 Effect of overexpression of histone H3 on the stability of mini-chromosome. Full size table Association of the 19S proteasome with centromeric chromatin Previous studies suggested that the proteasome (or its subcomplex) plays an important role in a variety of cellular processes, including DNA repair, regulation of gene expression and organelle regulation [33] , [34] , [35] , [36] , [37] . APIS (ATPases independent of 20S), a subcomplex of 19S RP, was shown to associate with various regions of the genome and regulate gene expression likely by remodelling chromatin [38] , [39] , [40] , [41] . We thereby tested if Rpt3 and other subunits of the proteasome associated with the centromeric chromatin. As shown in Fig. 4 , ChIP revealed that Rpt3 indeed associated with the centromeric chromatin. Furthermore, the analysis indicated that the mutant protein Rpt3-1 could maintain only a half of this activity ( Fig. 4a,b ) at both 26 and 36 °C. The level of Rpt3-1 mutant protein was slightly lower than the wild-type Rpt3 at 36 °C ( Fig. 4c ). A dramatic decrease in the activity of Rpt3-1 mutant protein to bind to centromeric chromatin at 36 °C ( Fig. 4b ) would partly be attributable to the lower level of the mutant protein in the extracts. We also performed immuprecipitation and found that the level of the wild-type Rpt3 protein co-precipitated with Cnp1 was much higher than that of the mutant Rpt3-1 protein ( Fig. 4d ). Other subunits of the proteasome were examined for their activity to associate with the centromeric chromatin. The results indicated that Rpt2/Mts2 and Rpn12/Mts3, both of which compose the 19S RP [42] , associated with the centromeric chromatin ( Supplementary Fig. 4a ). 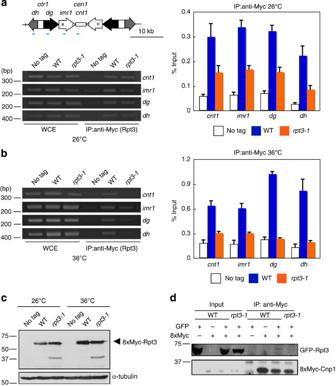Figure 4: Binding of Rpt3 to centromeric chromatin. (a,b) ChIP (left panels) and ChIP–qPCR (right panels) were performed with samples prepared from the strains expressing Rpt3 (WT) or the Rpt3-1 mutant protein (rpt3-1) tagged with 8xMyc, respectively, from the native promoter. The strains were grown at 26 °C (a) or 36 °C (b). All data represent the mean±s.e.m. (n=3). The blue bars indicate the position of primers used for ChIP. (c) The level of Rpt3 in the strains used inaandbwas examined by immunoblot. (d) Extracts were prepared from cells expressing Cnp1 tagged with 8xMyc and Rpt3 (WT) or the mutant Rpt3-1 (rpt3-1) tagged with GFP respectively, from the native promoter at 26 °C, and processed for immunoprecipitation by the antibody to Myc epitope. The asterisk indicates a band nonspecifically recognized by the antibody. Figure 4: Binding of Rpt3 to centromeric chromatin. ( a , b ) ChIP (left panels) and ChIP–qPCR (right panels) were performed with samples prepared from the strains expressing Rpt3 (WT) or the Rpt3-1 mutant protein ( rpt3-1 ) tagged with 8xMyc, respectively, from the native promoter. The strains were grown at 26 °C ( a ) or 36 °C ( b ). All data represent the mean±s.e.m. ( n =3). The blue bars indicate the position of primers used for ChIP. ( c ) The level of Rpt3 in the strains used in a and b was examined by immunoblot. ( d ) Extracts were prepared from cells expressing Cnp1 tagged with 8xMyc and Rpt3 (WT) or the mutant Rpt3-1 ( rpt3-1 ) tagged with GFP respectively, from the native promoter at 26 °C, and processed for immunoprecipitation by the antibody to Myc epitope. The asterisk indicates a band nonspecifically recognized by the antibody. Full size image We next tested if the 20S catalytic particle (CP) was involved in regulation of distribution of Cnp1. As shown in Supplementary Fig. 4b , α4,a subunit of the 20S CP, exhibited a significantly low activity to associate with the centromeric chromatin. The pts1 + gene encodes the β5 catalytic subunit of the 20S CP and a mutation ( pts1-727 ) causes a temperature sensitivity of cell growth at 36 °C [43] . Unlike the rpt3-1 mutant, gene silencing at cnt1 was not enhanced in the pts1-727 mutant ( Supplementary Fig. 5a ). Although the pts1 + gene encodes a product to play a central role in proteolysis, the level of Cnp1 in the pts1-727 mutant at the restrictive temperature was comparable with that of the wild-type strain ( Supplementary Fig. 5b ). The quantitative analysis by ChIP–quantitative PCR revealed that Cnp1 in the mutant was normally incorporated into cnt1 and imr1 . We however noticed that incorporation of Cnp1 into otr1 (represented by dg and dh ) was increased ( Supplementary Fig. 5c ). These results would suggest that although association of the 20S CP with the centromeric chromatin was not experimentally detectable, the 20S CP might regulate distribution of Cnp1 at otr1 (see Discussion). Requirement of Cut8 for proper distribution of Cnp1 Because both the centromere and proteasome are localized at the inner nuclear membrane (NM) in fission yeast [25] , [44] , we speculated that NM provides a site for association of 19S proteasome with the centromeric chromatin. To test this hypothesis, we examined the localization of the mutant protein Rpt3-1. As shown in Fig. 5a , we found the wild-type Rpt3 protein tagged with GFP on the rim of the nuclei as well as in the chromatin domain, thereby confirming localization of a fraction of the proteasome on NM. In contrast, the Rpt3-1 mutant protein tagged with GFP was found in the chromatin domain, but not on the rim ( Fig. 5a ), illustrating a defect of the Rpt3-1 protein in localization. These results would suggest that a failure of Rpt3-1 to localize on NM might be a major cause of the phenotypes. 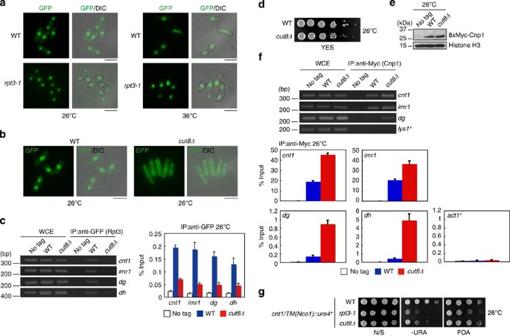Figure 5: Requirement of Cut8 for proper distribution of Cnp1. (a) The strains expressing GFP-tagged Rpt3 (WT) or the Rpt3-1 mutant protein (rpt3-1) from the native promoter were grown at 26 °C (left panel) or 36 °C (right panel) and observed under a fluorescence microscope. The bar indicates 10 μm. (b) The wild-type strain (WT) and a strain deleted for thecut8+gene (cut8Δ) expressing GFP-tagged Rpt3 (WT) from the native promoter were grown at 26 °C and observed under a fluorescence microscope. The bar indicates 10 μm. (c) Binding of Rpt3 to centromere 1 was examined by ChIP (left panel) and ChIP–qPCR (right panel). All data represent the mean±s.e.m. (n=3). (d) The wild-type strain (WT) and a strain deleted for thecut8+gene (cut8Δ) were spotted on YES media and incubated at 26 °C for 4 days. (e) The levels of Cnp1 tagged with 8xMyc (8xMyc-Cnp1) expressed from the native promoter was examined by immublot. (f) Distribution of 8xMyc-Cnp1 in centromere 1 was examined by ChIP (upper panel) and ChIP–qPCR (lower panel). All data represent the mean±s.e.m. (n=3). (g) The reporter geneura4+was integrated atcnt1 and examined its expression in each strain. Figure 5: Requirement of Cut8 for proper distribution of Cnp1. ( a ) The strains expressing GFP-tagged Rpt3 (WT) or the Rpt3-1 mutant protein ( rpt3-1 ) from the native promoter were grown at 26 °C (left panel) or 36 °C (right panel) and observed under a fluorescence microscope. The bar indicates 10 μm. ( b ) The wild-type strain (WT) and a strain deleted for the cut8 + gene ( cut8Δ ) expressing GFP-tagged Rpt3 (WT) from the native promoter were grown at 26 °C and observed under a fluorescence microscope. The bar indicates 10 μm. ( c ) Binding of Rpt3 to centromere 1 was examined by ChIP (left panel) and ChIP–qPCR (right panel). All data represent the mean±s.e.m. ( n =3). ( d ) The wild-type strain (WT) and a strain deleted for the cut8 + gene ( cut8Δ ) were spotted on YES media and incubated at 26 °C for 4 days. ( e ) The levels of Cnp1 tagged with 8xMyc (8xMyc-Cnp1) expressed from the native promoter was examined by immublot. ( f ) Distribution of 8xMyc-Cnp1 in centromere 1 was examined by ChIP (upper panel) and ChIP–qPCR (lower panel). All data represent the mean±s.e.m. ( n =3). ( g ) The reporter gene ura4 + was integrated at cnt 1 and examined its expression in each strain. Full size image Previous study showed that Cut8 serves as an anchor of the proteasome to NM [45] , [46] . In this study we found that Cut8 associated with the centromeric chromatin ( Supplementary Fig. 4a ). These results would suggest that Cut8 might link the proteasome, centromeres and NM. We thereby anticipated that introduction of a loss of cut8 + gene would release the proteasome from NM without affecting its function in proteolysis and allow to test if localization of the 19S proteasome on NM is a requirement for maintenance of proper distribution of Cnp1 in the centromeric chromatin. As shown in Fig. 5b , we confirmed release of Rpt3 from NM in a strain deleted for the cut8 + gene ( cut8Δ ). Rpt3 released from NM was unable to associate with the centromeric chromatin ( Fig. 5c ), demonstrating the importance of NM as a site for interaction between the proteasome and centromeric chromatin. We also found that the cut8 mutant was sensitive to ectopic expression of GFP-Cnp1, but not histone GFP-H3 ( Supplementary Fig. 6a ), and displayed multiple patches of GFP-Cnp1 in the nucleus, just like the rpt3-1 mutant ( Supplementary Fig. 6b ). Quantitative ChIP analysis revealed that the cut8 mutants, while growing normally at 26 °C maintaining the level of Cnp1 comparative with that of the wild-type strain Cnp1 ( Fig. 5d,e ), incorporated Cnp1 more actively into all three domains of the centromere, cnt1 , imr1 and otr1 ( Fig. 5f and Supplementary Fig. 6c ). Gene silencing at cnt1 was also enhanced ( Fig. 5g ). These results would suggest that the phenotypes associated with the rpt3-1 mutation were reproduced by simply releasing the proteasome from NM. In addition, for anchoring the proteasome to NM, the cut8 + gene product might be required for proteolysis and/or cell cycle regulation. We therefore attempted to test if the observed phenotype in the cut8 mutants (that is, abnormal distribution of Cnp1) was due to a failure in association of the proteasome to NM, but not to a defect in other processes in which Cut8 might be involved. A previous work demonstrated that the amino terminal 72 amino acids of Cut8 binds the proteasome [46] . We reasoned that overexpression of this fragment, designated Cut8(1–72), would mask the proteasome and interfere with the Cut8 to tether the proteasome to NM. Although overexpression of Cut8(1–72) in the wild-type strain did not cause growth defect or a decrease in the level of Rpt3 ( Fig. 6a,b ), it released the proteasome from NM in more than 40% of the cells ( Fig. 6c ). Quantitative ChIP analysis revealed that these cells incorporated Cnp1 more actively into all three domains of the centromere, cnt1 , imr1 and otr1 ( Fig. 6d ). Gene silencing at cnt1 was also enhanced ( Fig. 6e ). On the basis of these results, we would propose that association of the proteasome to NM mediated by Cut8 is a crucial requirement for regulation of distribution of Cnp1 at the centromere. 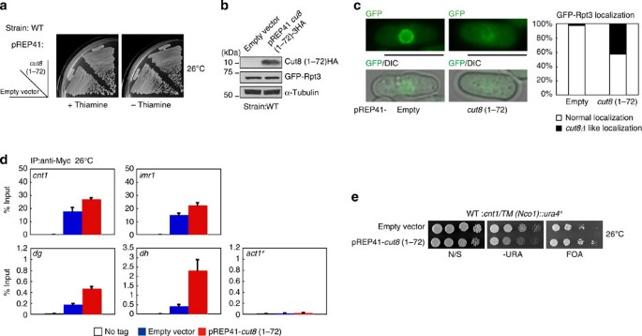Figure 6: Effect of overexpression of Cut8(1–72) on distribution of Cnp1. The wild-type strain was transformed with an empty vector or a plasmid allowing overexpression of Cut8(1–72) tagged with HA epitope in the absence of thiamine. The transformants were examined for their growth (a), levels of Cut8(1–72) and Rpt3 (b), localization of the GFP-Rpt3 (c), distribution of Cnp1 in the centromeric chromatin (d) and gene silencing atcnt1(e). The bar indicates 10 μm. All data represent the mean±s.e.m. (n=3). Figure 6: Effect of overexpression of Cut8(1–72) on distribution of Cnp1. The wild-type strain was transformed with an empty vector or a plasmid allowing overexpression of Cut8(1–72) tagged with HA epitope in the absence of thiamine. The transformants were examined for their growth ( a ), levels of Cut8(1–72) and Rpt3 ( b ), localization of the GFP-Rpt3 ( c ), distribution of Cnp1 in the centromeric chromatin ( d ) and gene silencing at cnt1 ( e ). The bar indicates 10 μm. All data represent the mean±s.e.m. ( n =3). Full size image In this study by characterizing the phenotypes of the rpt3-1 and cut8 mutants, we have elucidated a role of the proteasome (or its subcomplex) in regulating distribution of CENP-A by associating with centromeric chromatin. We speculate that the chromatin state at the centromere in the rpt3-1 mutant is altered at least in two aspects. First, the cnt and imr domains contain more Cnp1 in the mutant. Similarly, the otr domains, which are normally a Cnp1-poor region, contain Cnp1. These observations would suggest that the ratio of Cnp1-nucleosomes to H3-nucleosomes and/or the density of the total nucleosomes at cnt and imr domains would be higher in the mutant. Second, the cnt domains of the mutant contain Swi6. The presence of Swi6, a heterochromatin binding protein, at cnt domains suggests that the cnt -chromatin might be heterochromatinized. These changes both in quantity and quality of centromeric chromatin would be a main cause of the enhanced gene silencing and the instability of the mini-chromosome Ch16. The heterochromatinization and/or dense distribution of nucleosomes would make centromeric chromatin stiffer and prevent proper ‘stretch’ of the centromere to sense tension for accurate chromosome segregation [47] , [48] . A recent study has reported that the 19S proteasome regulates gene expression by evicting nucleosomes in budding yeast [49] . We propose that a similar activity of the 19S proteasome eliminates CENP-A or CENP-A containing nucleosomes and maintains proper distribution of CENP-A around the centromere. Although speculative, the six ATPases (Rpt1–Rpt6) in 19S RP may be directly responsible for eviction of the nucleosomes. Alternatively, a fraction of 19S RP partnered by a histone chaperon might be specialized for eviction. The FACT and HIRA histone chaperones are co-immunoprecipitated with the ATPases, Rpt6 and Rpt3, respectively [38] , [50] . The latter study has employed liquid chromatography-tandem mass spectrometry and demonstrated that the 19S subunit of the proteasome is reproducibly co-purified with Slm9, a subunit of HIRA. Although the 19S RP has been proposed to exist as a protein complex physically independent from the 20S CP and perform non-proteolytic functions in regulation of gene expression [39] , [49] , [51] , a recent report has shown that in budding yeast, the 19S RP is recruited together with the 20S CP to transcriptionally active chromatin [52] . Requirement of the 20S CP for regulation of gene expression is therefore currently under debate. Our analysis has indicated that incorporation of Cnp1 is increased at otr1 , but not at cnt1 or imr1, in the pts1-727 mutant that carries mutation in the gene encoding the β5 catalytic subunit of the 20S CP. Distribution of Cnp1 at the otr domain might require a proteolytic activity of the proteasome, though a relevant substrate is to be identified. We would therefore not exclude a possibility that some of the phenotypes associated with the rpt3-1 mutation could be caused indirectly due to a defect in a proteolytic function of the proteasome. Further investigation is obviously required to clearly define the role of the proteasome in regulation of distribution of Cnp1/CENP-A. Because the level of Cnp1 in the rpt3-1 and cut8 mutants is comparable with that in the wild-type strain, excessive incorporation of Cnp1 in the centromeric chromatin is not due to a defect in degradation of Cnp1. We would speculate that by associating with the centromeric chromatin with the aid of Cut8, the proteasome is responsible for eliminating excess chromatin-bound Cnp1. A single CENP-A nucleosome functions as the centromere in budding yeast [53] , suggesting that promiscuous incorporation of CENP-A in chromatin would be an immediate risk of neocentromere formation. To avoid the risk, the proteasome is responsible for degrading excess CENP-A in this organism [54] , [55] . Our study has demonstrated a role of the proteasome in preventing spread of CENP-A in the centromere. Because the spread of CENP-A would possibly enhance a chance for the centromere to slide from the original position, the proteasome might play a role as an antagonist of ‘centromere repositioning’, the evolutionary movement of the centromere along the chromosome without marker order variation [56] . Strains, culture media and strain construction An S. pombe haploid wild-type strain 972 ( h − ) and its derivatives used in this study are listed in Supplementary Table 2 with the source/origin. The culture media were complete YES, MEA sporulation medium and minimal EMM2 (ref. 57 ). The cell number was measured using a haematology analyser (Sysmex F-520P). To construct a strain expressing 8xMyc-tagged Cnp1, the PCR-based standard method [58] was followed. The open reading frame of the cnp1 + gene was replaced with the hphMX6 cassette containing 8xMyc-Cnp1. A strain expressing Rpt3 tagged with GFP was constructed with a similar strategy. A strain expressing GFP-tagged Cnp1 from the nmt promoter was constructed by integrating a plasmid that contained the nmt1 GFP-cnp1 + construct. All integrants were examined for their integrated locus by PCR as well as crossing. Western blotting Cell extracts were prepared from exponentially growing S. pombe cells. The cells suspended in lysis buffer (50 mM HEPES (pH 7.5), 150 mM NaCl, 1 mM MgCl 2 , 1 mM EDTA (pH 7.5), 0.1% NP-40, 2 mM PMSF, protease inhibitor cocktail (SIGMA)) were disrupted by Bead Smash 12 (WAKENYAKU) at 4 °C. After centrifugation, the supernatants were used for SDS–polyacrylamide gel electrophoresis (SDS–PAGE). The extracts were separated by SDS–PAGE gel and blotted to nitrocellulose membranes. Antibodies for western blotting were diluted as follows: mouse anti-GFP (Roche) 1:1,000; anti-Myc (9E10, Calbiochem) 1:1,000; anti-H3 (1791, abcam) 1:1,000; anti-HA (12CA5, Roche) 1:3,000; and TAT1 anti-α-tubulin (gift from K. Gull, Oxford, UK) 1:5,000. Blots were developed using ECL reagents (Substrate Plus (Pierce), ECL prime (GE Healthcare). Full scan of western blotting shown in Figs 2b , 4c and 5e are shown in Supplementary Fig. 7 . TCA precipitation Cell extracts were prepared by the trichloroacetic method (TCA precipitation) for analysis of Cnp1. TCA solution (100%) was added to cell cultures at a final concentration of 20%, and cells were collected by centrifugation at 4 °C. Harvested cells were crushed in 10% TCA solution using glass beads and Bead Smash 12 (WAKENYAKU), and proteins were precipitated by centrifugation at 14,000 × g for 15 min at 4 °C. Precipitates were boiled in 1X LDS buffer (Invitrogen) with 0.16 M Tris and β-mercaptoethanol at 70 °C for 10 min. Boiled samples were centrifuged at 15,000 × g for 5 min to remove cell debris and quantified using a Bradford Assay Kit (Bio-Rad). Microscopy S. pombe strains were grown in YES or EMM2 medium. All images were acquired on a LEICA DM5500B (Leica) microscope equipped with a HAMAMATSU ORCA-ER camera. Colony spotting assay The cells were grown to logarithmic phase in YES medium, then the cells were serially diluted from 1 × 10 7 to 1 × 10 3 cells ml −1 (10-fold dilution), and 5 μl of each was spotted onto YES plates. For centromere silencing assay, 5-fold dilution of the cells were spotted onto N/S plates (EMM+leucine+adenine+uracil), –URA plates (N/S lacking uracil) and FOA plates (N/S+1 mg ml −1 5′-FOA). Mini-chromosome stability assay The stability of mini-chromosome was determined by a method developed by Allshire et al. [59] First, the cells were plated on YE (for Table 1 ) or EMM containing 10 μg ml −1 adenine (for Table 2 ) to determine the initial percentage of the cells carrying the mini-chromosome. After incubation in the non-selective medium (Ade + ), the final percentage of the cells carrying the mini-chromosome was determined. The rate of mini-chromosome loss per division was estimated using the formula: loss rate=1−(F/I) 1/N (F, the final percentage of cells carrying mini-chromosome; I, the initial percentage of cells carrying mini-chromosome; N, the number of generations between F and I) Immunoprecipitation Approximately 10 8 cells were spheroplasted according to Masumoto et al. [60] with modifications. Cells were incubated at room temperature for 5 min in SP1 buffer (1.2 M D-sorbitol, 50 mM citrate-phosphate (pH5.6), 10 mM dithiothreitol), followed by incubation for 30 min at 36 °C with SP2 bufer (1.2 M D-sorbitol 50 mM citrate-phosphate (pH 5.6) containing 20 mg ml −1 lyzing enzymes (SIGMA)). The resulting spheroplasts were washed twice with a buffer (20 mM HEPES-KOH (pH 7.5), 0.4 M sorbitol, 150 mM sodium acetate, 2 mM magnesium acetate), followed by incubation with the cross-linking buffer (20 mM HEPES-KOH (pH 7.5), 0.4 M sorbitol 150 mM sodium acetate, 2 mM magnesium acetate, 2 mM dithiobis (succinimidyl propionate (DSP; Pierce)) for 30 min at room temperature. The reaction was terminated by incubation for 5 min with 50 mM Tris-HCl (pH 7.5). After the cross-linking treatment, the procedure was carried out according to Kawashima et al. [61] with modifications. Cells were washed with lysis buffer 1 (20 mM HEPES-KOH (pH 7.5), 140 mM NaCl, 1 mM EDTA (pH 7.5)) and then resuspended in lysis buffer 2 (buffer 1 containing 1% Triton X-100, 1 mM PMSF and protease inhibitor cocktail (SIGMA)). The spheroplasts were lysed by Bead Smash 12 (WAKENYAKU). Crude cell extracts were sonicated six times (10 s each time), and the supernatant was collected by centrifugation. Cell extracts were incubated with 10 μl of the antibody to the Myc epitope (sc-40; SANTA CRUZ) for immunoprecipitation for 6 h at 4 °C. After washing, the immunoprecipitates were analysed by SDS–PAGE followed by western blotting. The antibody to the Myc epitope (9E10, Calbiochem) was diluted to 1:500 and the antibody to GFP (Roche) to 1:250. Chromatin Immunoprecipitation (ChIP) assay Exponentially growing cells (5 × 10 8 cells) were fixed with 1% formaldehyde for 60 min. The reaction was then quenched by adding 330 mM final concentration of glycine to the culture and incubating for 5 min. The cells were collected by centrifugation and washed three times with PBS. Cell lysates were prepared by glass beads vortexing in FA-lysis buffer (50 mM HEPES-KOH (pH7.5), 150 mM NaCl, 1 mM EDTA, 0.1% sodium deoxycholate, protease inhibitor cocktail (SIGMA), 1 mM PMSF) containing 0.5% SDS. After discarding the glass beads, the cross-linked chromatin was pelleted by centrifugation at 12,000 × g for 20 min at 4 °C, washed once with FA-lysis buffer containing 0.1% SDS. After that, the pellet was resuspended in the same buffer and sonicated using Bioruptor (Cosmo Bio) at 4 °C to yield fragments with average size of 500 bp. The sonicated sample was clarified by centrifugation at 12,000 × g for 20 min at 4 °C. The resultant soluble chromatin solution was supplemented with 1% Triton X-100. ChIP assay was performed by applying mouse anti-GFP (Roche), anti-Myc (9E10, Calbiochem) to the chromatin solution for 2 h at 4 °C, followed by overnigtht incubation with Protein A (or Protein G)-conjugated Dynabeads (Invitrogen) at 4 °C. The beads were washed three times in FA-lysis buffer containing 0.1% SDS and 1% Triton X-100; once in the same buffer containing 0.5 M NaCl; once in 10 mM Tris-Cl (pH8.0), 250 mM LiCl, 1 mM EDTA, 0.5% NP-40 and 0.5% sodium deoxycholate; once in TE. To elute DNA and revert cross-linking, the beads were incubated with SDS-TE (TE containing 1% SDS) for 15 h at 65 °C, followed by digestion with proteinase K (Merck) for 2 h at 42 °C. After extraction with phenol and phenol-chloroform-isoamyl alcohol, DNA was precipitated with isopropanol in the presence of glycogen and suspended in TE. ChIP analysis was performed by quantifying the amount of DNA in ChIP and whole extract samples (WCE), using MyiQ2 (Bio-rad). ChIP DNA amount relative to WCE was determined by calculating their Ct value difference. For ChIP of the components of the proteasome, cross-linking was performed by treatment of 10 mM dimethyl adipimidate (DMA; Thermo) and 1.5% formaldehyde as described [62] for 60 min. The ChIP on-chip analysis was performed accordingly to a procedure developed by Ishii et al. [19] . ChIP-purified DNA and DNA of soluble chromatin input (WCE) were treated with 10 μg ml −1 RNase A (Sigma), flush-ended using T7 DNA polymerase (New England Biolabs) and ligated with the double-stranded DNA linker JW102/JW103 using T4 DNA ligase (New England Biolabs). Each DNA was amplified using AmpliTaq DNA polymerase (Applied Biosystem) and JW102. The amplified ChIP and WCE were labelled with Cy5-dUTP and Cy3-dUTP (Agilent Technologies), repectively, by using the Agilent Genomic DNA Labelling Kit Plus (Agilent Technologies). Hybridization was carried out at 65 °C for 40 h against the 4 × 44 K slide of S. pombe whole genome ChIP on chip microarray (Agilent Technologies) according to the manufacturer’s instructions. The slide was then washed with Wash buffer 1 for 5 min at room temperature and with Wash buffer 2 for 5 min at 31 °C according to the manufacturer’s instructions (Agilent Technologies), in ozone-depleted surroundings. Finally, the array slide was scanned using the Agilent Microarray Scanner G2505B and Scan Control Software G2565BA, followed by extraction of information from the pombe features using Feature Extraction Software 9.5.1.1 (Agilent Technologies). For each data set, intra-array Lowess (intensity-dependent) normalization was performed using the ChIP Analysis Software 1.3.1 (Agilent Technologies), and the enrichment ratios were calculated by dividing the normalized ChIP (Cy5) signals against WCE (Cy3) signals. The nucleotide sequences of the primer sets used in this study are listed in Supplementary Table 1 . Isolation of the rpt3-1 mutant A wild-type strain carrying pREP41-GFP- cnp1 + was chemically mutagenized according to Matsumoto and Beach [63] . NTG (N-methyl-N′-nitrosoguanidine) was employed to mutagenize SP6 (wild-type strain), which carried pREP41- cnp1 in the leu1-32 background. Exponentially grown cells suspended in TM buffer (50 mM Tris malate (pH 6.0)) were treated with NTG (500 μg ml −1 ) at 26 °C for 20 min and washed three times with TM buffer. Cells were grown in the YES liquid medium for 4 h at 26 °C and washed with EMM2 medium containing thiamine. Cells were grown in the same medium for 4 h at 26 °C. The survivors were plated on the EMM2 plates containing thiamine and grown at 26 °C. They were subsequently transferred onto EMM2 plates with and without thiamine by replica and grown at 36 °C. The strains that exhibited temperature sensitivity only when GFP-Cnp1 was expressed were selected. They were then individually examined under a fluorescence microscope. We stored mutants with abnormal distribution of GFP-Cnp1 in the nucleus. Tetrad analysis indicated that five strains including the rpt3-1 mutant carried a single mutation responsible for the phenotypes (temperature sensitivity and abnormal distribution of GFP-Cnp1). Isolation of the rpt3 + gene By using the temperature sensitivity as a selection marker, a genomic DNA fragment complementing the temperature sensitivity was isolated from a fission yeast genomic DNA library. The integration mapping proved that this fragment originated from the rpt3-1 locus. A PCR-based strategy was used to identify the mutation site within the rpt3 + coding sequence. The rpt3-1 mutant gene contained nonsense mutation of Q384. Accession code : Microarray data have been deposited in the Gene Expression Omnibus (GEO) data base with the accession no. GSE44594 . How to cite this article: Kitagawa, T. et al. The 19S proteasome subunit Rpt3 regulates distribution of CENP-A by associating with centromeric chromatin. Nat. Commun. 5:3597 doi: 10.1038/ncomms4597 (2014).